Carbon storage and potential methane production in the Hudson Bay Lowlands since mid-Holocene peat initiation Peatlands have influenced Holocene carbon (C) cycling by storing atmospheric C and releasing methane (CH 4 ). Yet, our understanding of contributions from the world’s second largest peatland, the Hudson Bay Lowlands (HBL), Canada, to peat-climate-C-dynamics is constrained by the paucity of dated peat records and regional C-data. Here we examine HBL peatland development in relation to Holocene C-dynamics. We show that peat initiation in the HBL is tightly coupled with glacial isostatic adjustment (GIA) through most of the record, and occurred within suitable climatic conditions for peatland development. HBL peatlands initiated most intensively in the mid-Holocene, when GIA was most rapid and climate was cooler and drier. As the peat mass developed, we estimate that the HBL potentially released 1–7 Tg CH 4 per year during the late Holocene. Our results indicate that the HBL currently stores a C-pool of ~30 Pg C and provide support for a peatland-derived CH 4 contribution to the late Holocene atmosphere. Peatlands are an important component of the global carbon (C) cycle, as long-term atmospheric C dioxide (CO 2 ) sinks and methane (CH 4 ) sources. Holocene peat accumulation in northern high latitudes occurs under cool, humid conditions. The storage of atmospheric C in peatlands, as partially decomposed vegetation, has resulted in a net long-term climatic cooling. Quantifying the influence of peatland development in the global C-climate system necessitates refined estimates of peatland extent and development in relation to paleoclimate, peat C accumulation and long-term potential atmospheric CO 2 and CH 4 dynamics [1] , [2] . A key uncertainty stems from the paucity of detailed peatland age and C records from the world’s second largest continuous peatland, the Hudson Bay Lowlands (HBL), Canada. HBL peatlands are assumed to be a globally significant C-pool, and peatland development in this region is potentially driven by both glacial isostatic adjustment (GIA) and climate. However, these hypotheses remain untested at the regional scale and have never been supported by a larger data set. Before peatland initiation in the HBL, subsidence in excess of 200 m following the final collapse of the Laurentide ice sheet, resulted in inundation of the region by the post-glacial Tyrrell Sea [3] until ~8.5 ky. Since this time, land has been emerging from the Hudson and James Bays at GIA rates that are among the fastest globally [4] , [5] , [6] . Today, a nearly continuous peat cover over low relief deposits of glacio-marine sediments [7] stretches from the shoreline of Hudson and James Bays inland to the margin of the upland Precambrian Shield. Based upon available land classification data [8] , peat accumulating features, dominated by bogs and fens, occupy up to 90% of the HBL’s 372,000 km 2 landscape [7] , [8] , [9] or ~10% of the northern peatland area [10] , [11] . Permafrost is estimated to occur in ~1% of the HBL [8] , [9] , principally as continuous permafrost along the Hudson Bay coast [8] , and as sporadic to discontinuous permafrost in the southern and central HBL, respectively [9] . The HBL’s climate is microthermal, influenced by Arctic air masses, strong winds and ice cover on the Hudson Bay. Modern average climate (1971–2000) is characterized by a mean annual temperature (MAT) of −2.5±1.8 °C and a mean growing season temperature of 10.8±1.0 °C over a period of 119–162 days [12] . Total annual precipitation ranges from 430 to 740 mm with half to two-thirds of the precipitation occurring during the growing season [12] . Since deglaciation, northern peatlands have accrued 500±100 Pg C (refs 1 , 10 , 13 ), equivalent to 100–200 p.p.m.v. atmospheric C dioxide (CO 2 ) [14] . However, northern wetlands, and especially minerotrophic peatlands [15] , [16] , are one of the strongest natural sources of methane, and release 21–43 Tg CH 4 per year to the atmosphere [17] , [18] . Atmospheric CH 4 concentrations are mostly source-driven [18] , [19] , and peatland C-dynamics can account for part of this variation [6] , [8] , [9] , [10] . Polar ice-core records reveal that atmospheric CH 4 concentrations rose twice during the Holocene: first in the early Holocene during a period of continental deglaciation (11.6–8 ky before present (BP)); and second, during the mid- to late Holocene (5 ky BP—present), following a brief decline in atmospheric CH 4 (ref. 20 ). Although subject to large uncertainties, inter-hemispheric CH 4 gradients suggest that northern terrestrial wet ecosystems, including peatlands can explain a portion of the variability in atmospheric CH 4 during both the early and late Holocene [13] , [15] , [21] . Examination of the dynamic coupling between peatland development and Holocene atmospheric CH 4 variability may provide additional insight into long-term peatland-climate-C dynamics. During the early Holocene, high insolation and seasonality coupled with the availability of newly exposed surfaces following deglaciation, resulted in a tripling of peatland extent and precursor wetland conditions. Thus, post-glacial wet and reducing conditions together with rapid peatland expansion during the early Holocene are associated with rising atmospheric CH 4 concentrations [15] , [16] . However, global syntheses of available northern peatland initiation dates have shown lower rates of peatland expansion after 9 ky BP, further implying reduced peatland-derived CH 4 contributions to the mid- and late Holocene atmospheres [13] , [15] . However, given limited detailed evidence from spatially extensive and late emerging peatlands such as the HBL, quantification of the potential contribution of northern peatlands to the late Holocene CH 4 rise has not been fully possible [11] , [21] . Although northern peatlands could contribute in part to the rise in CH 4 in the late Holocene, potential alternative terrestrial sources may include early anthropogenic activity, such as rice cultivation, biomass burning and deforestation [22] , lateral expansion of existing high-latitude peatlands [23] , permafrost dynamics [10] and/or contributions from tropical wet ecosystems [13] , [19] . Here, we report on the history of peat development in the HBL, using a synthesis of peat ages and detailed peat C records. With these new data, we examine the relationship between climatic and geophysical controls relative to peatland initiation and expansion in the HBL and evaluate the possible connection between HBL peatland development and atmospheric C dynamics, during the Holocene. Our evidence supports the hypothesis of potential peatland-derived CH 4 emissions during the late Holocene, and fills a key gap in determining the potential contribution of northern peatlands to late Holocene atmospheric CH 4 concentrations. Although climate has been invoked as the dominant control on northern peatland initiation [15] , [16] , [24] , GIA appears to be an even more fundamental control of peatland initiation and expansion in the dynamic landscape of the HBL [4] , [25] , [26] . We estimate that HBL peatlands have accumulated a globally significant peat C pool of ~30 Pg C over the Holocene. During the most intense period of peat initiation between 4 and 7 ky calendar years BP (cal BP), thin peat profiles over marine sediments may limit the potential for CH 4 emission, because of the possible influence of marine pore waters driving sulfate reduction [27] , [28] and the prevailing cold, dry climate inferred from a landscape-scale pollen reconstruction (northern Quebec) [29] . However, by 3 ky cal BP peatlands with a mean thickness of 1 m occupied 80% of the HBL’s current extent, and were developing under climatic conditions similar to today [29] , supporting a potential CH 4 emission of 1–7 Tg CH 4 per year. Acknowledging the complexity of atmospheric CH 4 dynamics, a potential late Holocene CH 4 emission of this magnitude from the HBL cannot alone explain the late Holocene rise in global atmospheric CH 4 concentrations. Still, our new estimates provide evidence that peatland development in the HBL may constitute a potential CH 4 contribution to late Holocene atmosphere that should be accounted for alongside other prospective anthropogenic and natural terrestrial CH 4 sources in global C budgets. GIA and paleoclimate as controls of HBL peatland dynamics Today, land is emerging at a rate of 5–12 mm per year in the HBL [4] , with maximum isostatic uplift rates centered near the north-west and south-east reaches of the landscape ( Fig. 1 ). 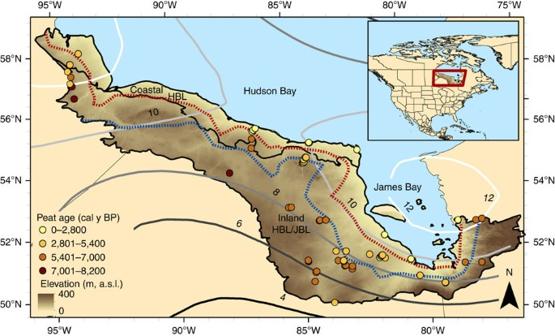Figure 1: Holocene land emergence and peatland expansion in the Hudson Bay Lowlands. The physiographic region of the Hudson Bay Lowlands (HBL), Canada, includes the coastal HBL (Coastal) and the inland HBL and James Bay Lowland (Inland HBL/JBL) ecoregions58. Contours (grey gradient) represent modern isostatic uplift rates (mm per year)4, whereas brown shading represents modern surface elevation (m, above sea level) generated using 1:250K Canadian digital elevation data70. The 5.5-ky (blue dashed) and 3.0-ky (red dashed) paleo-coasts presented here were extracted from the paleotopography database4,61. Peatland study locations are colour-coded by basal14C ages and grouped according to trends in peat initiation frequency (Supplementary Table 1). Our synthesis of 33 new and 67 previously reported peat ages ( Supplementary Table 1 ) documents the spatio-temporal variability in peat initiation and expansion in the HBL, following retreat of the Laurentide ice sheet. The mean and standard deviation depth of peat is 203±89 cm and the median basal age is 5 ky cal BP for this series of peat records, whereas the oldest basal date returned was 8.2 ky cal BP recovered from the margin of inundation by the post-glacial Tyrrell Sea. It provides an oldest minimum peat age for the peatlands of the HBL. Figure 1: Holocene land emergence and peatland expansion in the Hudson Bay Lowlands. The physiographic region of the Hudson Bay Lowlands (HBL), Canada, includes the coastal HBL (Coastal) and the inland HBL and James Bay Lowland (Inland HBL/JBL) ecoregions [58] . Contours (grey gradient) represent modern isostatic uplift rates (mm per year) [4] , whereas brown shading represents modern surface elevation (m, above sea level) generated using 1:250K Canadian digital elevation data [70] . The 5.5-ky (blue dashed) and 3.0-ky (red dashed) paleo-coasts presented here were extracted from the paleotopography database [4] , [61] . Peatland study locations are colour-coded by basal 14 C ages and grouped according to trends in peat initiation frequency ( Supplementary Table 1 ). Full size image Spatially associating basal peat age inventories with post-glacial land emergence histories reveals that peat initiation in the HBL was tightly coupled with GIA ( Fig. 2 ). The theoretical rate of GIA decays exponentially with time, hence, the fastest rates of isostatic uplift occur immediately following deglaciation [4] . Likewise, new peatland initiation in the HBL also appears to decline through time, with the greatest rates of peat initiation in the HBL recorded during the period 4–7.5 ky cal BP, referred to here as the mid-Holocene ( Fig. 2 ). A small bias towards sampling older, deeper peatlands may contribute to the apparent reduction in the rate of peat initiation events later in the Holocene. However, we expect that a gridded sampling strategy across the entire HBL would reveal a comparable temporal pattern because of increasingly smaller additions of new land with time, as a result of long-term exponentially declining rates of GIA in the HBL. Thus, a potential sampling bias towards deeper peatlands does not undermine our conclusions. 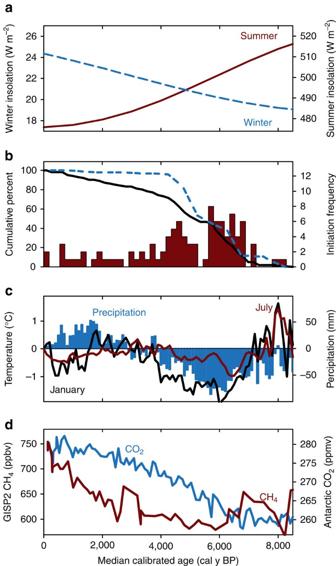Figure 2: Peat initiation dynamics in the Hudson Bay Lowlands. (a) Winter (blue dashed) and summer (red solid) insolation during last 8.5 ky at 60 °N (ref.57). (b) Frequency of post-glacial peatland initiation (red histogram) in the Hudson Bay Lowlands, Canada, inferred from basal radiocarbon dates (n=100, mean 2σage range bins), cumulative peatland initiation (%;n=100; black solid) and corresponding cumulative land emergence (%,n=100; blue dashed). Here, the timing of land emergence, driven by the exponential decay in glacial isostatic adjustment, is spatially related to each peat record included in this study. Using the geographic coordinates for each peat record, the corresponding time of land emergence was extracted from a paleotopography data set4,61. The cumulative land emergence and peat initiation curves presented here are directly related and can be compared for the purpose of examining lags between the timing of land emergence and the timing of peat initiation at specific peatland sites (refer toFig. 1for total surface area estimates through time using the paleo-coasts). (c) Reconstruction of January (black) and July (red) temperature and annual precipitation (blue bars) anomalies from the North American Pollen Database (Northern Quebec pollen region)29; and (d) GISP2 (Greenland) ice core record of atmospheric methane (CH4) concentration20(red) and Antarctic ice core record of atmospheric carbon dioxide (CO2) concentrations59(blue) during the Holocene. Figure 2: Peat initiation dynamics in the Hudson Bay Lowlands. ( a ) Winter (blue dashed) and summer (red solid) insolation during last 8.5 ky at 60 °N (ref. 57 ). ( b ) Frequency of post-glacial peatland initiation (red histogram) in the Hudson Bay Lowlands, Canada, inferred from basal radiocarbon dates ( n =100, mean 2 σ age range bins), cumulative peatland initiation (%; n =100; black solid) and corresponding cumulative land emergence (%, n =100; blue dashed). Here, the timing of land emergence, driven by the exponential decay in glacial isostatic adjustment, is spatially related to each peat record included in this study. Using the geographic coordinates for each peat record, the corresponding time of land emergence was extracted from a paleotopography data set [4] , [61] . The cumulative land emergence and peat initiation curves presented here are directly related and can be compared for the purpose of examining lags between the timing of land emergence and the timing of peat initiation at specific peatland sites (refer to Fig. 1 for total surface area estimates through time using the paleo-coasts). ( c ) Reconstruction of January (black) and July (red) temperature and annual precipitation (blue bars) anomalies from the North American Pollen Database (Northern Quebec pollen region) [29] ; and ( d ) GISP2 (Greenland) ice core record of atmospheric methane (CH 4 ) concentration [20] (red) and Antarctic ice core record of atmospheric carbon dioxide (CO 2 ) concentrations [59] (blue) during the Holocene. Full size image Available paleoclimate data [29] , [30] for the entire period of Holocene peatland development in the HBL indicate that climatic conditions were continuously suitable for peatland development [11] . However, the coldest winters and summers together with the period receiving the least precipitation occurred between 4 and 7 ky cal BP, synchronous with both the highest rates of peat initiation and emergence of new land available for paludification. Declining rates of peat initiation up to and during the period of Neoglacial cooling (~2 ky cal BP) were associated with cooler temperatures and more precipitation based upon regional pollen-based paleoclimatic reconstructions ( Fig. 2c ) [29] . Contemporary climate in the HBL likely varies spatially, because of the seasonal influence of the Hudson Bay. However, few paleoclimatic records are available for the HBL, restricting examination of regional climate variation on peatland initiation and C dynamics during the Holocene. HBL C storage and potential Holocene CH4 emissions The physiographic region of the HBL is composed of two main ecoregions, which differ in terms of spatial extent, peat age and depth, and C-storage capacity. The more recently emerged coastal HBL ecoregion accounts for 62,370 km 2 , whereas the inland HBL and James Bay Lowland (JBL) ecoregions together account for 309,350 km 2 . Coastal HBL peatlands included in this study are occupied by thin peat deposits, with a median peat depth of 58 cm and a mean peat age of 1,900±1,830 cal y BP ( n =13). By contrast, the inland HBL peatlands studied here have a median peat depth of 218 cm and a mean peat age of 5,220±1,450 cal y BP ( n =86). We estimated the total C pool for the HBL peatland complex and for each of the two principal ecoregions, based upon peat age and C content. Our results reveal a mean areal C mass of 89±27 kg C m −2 ( n =100) for the HBL that accumulated at a mean rate of 18.5±5.7 g C m −2 y −1 and has a mean C-density of 0.05±0.01 g cm −3 . Multiplication of the mean total peat C mass by the total peatland surface area of 334,800 km 2 results in an HBL C pool of approximately 30 Pg C (29–31 Pg C). Permafrost occupies a relatively small fraction of the HBL, and although our record proportionally includes permafrost features, possible variation in C-mass from permafrost-impacted peatlands could not be adequately assessed here because of sample limitations. However, we considered variation in areal C mass between the inland and coastal ecoregions. We found that the median C mass was significantly greater ( U =107, P <0.001) inland (99 kg m −2 ) than near the coast (40 kg m −2 ).Taking this difference into consideration yields an area-weighted total C pool of ~27.6 Pg C for the inland HBL/JBL ecoregions and ~2.2 Pg C for the coastal ecoregion. Modern seasonal CH 4 fluxes range from 1 to 50 g CH 4 m −2 y −1 for peatlands in the HBL [31] , [32] , [33] , [34] , with scaled-up areal emissions ranging from 5 to 20 g CH 4 m −2 y −1 for the HBL region [35] , [36] , as defined here. Although peatland CH 4 fluxes are highly uncertain, we use the latter, more conservative regional CH 4 flux range to estimate the potential CH 4 contributions from the HBL to the mid- and late Holocene atmosphere. Given a 5.5-ky cal BP HBL landscape, we find that peat could cover 50% of the modern HBL extent, with a mean peat depth of 33 cm, and could potentially emit 0.7–3.7 Tg CH 4 per year. Climate at this time was colder and drier than today ( Fig. 2c ) [29] , and CH 4 emissions may have stemmed from the terrestrial–aquatic interface. However, areas with thin peat in contact with marine sediments, as evidenced by the occurrence of salt marsh vegetation remains near the peat-mineral interface [37] , may conversely experience reduced potential CH 4 flux, due in part to interactions with marine pore and surface waters [27] , [28] . By contrast, a 3-ky cal BP HBL peatland landscape could occupy approximately 80% of the modern peatland surface area, with a mean peat thickness of 1 m. The accrual of a thick peat mass could limit the influence of the marine sediments upon late Holocene peatland dynamics. Accordingly, a 3-ky cal BP peatland extent, operating under climatic conditions similar today (as indicated by the regional paleoclimate record), could support a potential CH 4 flux of 1.2–6.8 Tg CH 4 per year to the late Holocene atmosphere. Given a unit conversion factor 2.78 Tg CH 4 p.p.b. −1 and a 8.4-y CH 4 lifetime [18] , [19] , the potential CH 4 emissions from the HBL during the late Holocene could account for an increase of 4–21 p.p.b. We used a landscape scale estimate of snow-free CH 4 flux for the geographic extent of the HBL, according to the spatial extent described here. Estimates from static chamber measurements are subject to large seasonal to inter-annual variability, and if considered alone may predict reduced potential CH 4 emissions at the local scale [32] , [34] or enhanced potential CH 4 flux up to six times greater than these regional scale emission rates [38] , [39] . Our synthesis confirms that peat initiation in the HBL began several millennia later than many northern peatland regions, including the extensive peatlands of western Canada and Siberia. Two periods of intensified peat initiation are evident during the mid-Holocene. The first occurred between 5.6 and 7 ky cal BP, as new land emerged from the Tyrrell Sea approximately four times faster than the modern rate of isostatic uplift [26] . Following an ~0.6 ky apparent gap in peat initiation, a second phase of intensified peat initiation occurred between 4.2 and 5 ky cal BP ( Fig. 2 ), when isostatic uplift was approximately three times faster than today. Although the gap between the two most intense periods of initiation in the HBL may be due to a lack of available peat records in this data set, other studies have attributed similar peat initiation gaps to the occurrence of large-scale drainage events. In the HBL, regional drainage events resulting from outbursts of dammed water features or uplift-mediated changes in stream flow paths have been documented [25] , [40] . Half of the peatlands examined here initiated synchronously with land emergence from the post-glacial Tyrrell Sea ( Fig. 2b ). However, comparison of cumulative peat initiation and post-glacial land emergence curves reveal a divergence after 5.8 ky cal BP, suggesting a time lag between emergence of available land and establishment of peat-accumulating features on the parcels of newly emerged land. This apparent temporal lag in peat initiation relative to the emergence of the corresponding parcel of land appears to have continued until present. Syntheses of North American peat initiation records have reported lags between land emergence and peat initiation of up to 4 ky throughout the Holocene, which have been attributed in part to the slow migration of peatland plant propagules to the newly emerging surface [41] . However, in the HBL, peat-forming vegetation appears to have rapidly established on the newly emerging land between 5.6 and 7 ky cal BP, thus the slow migration of peatland plant propagules does not adequately account for the time lag between land emergence and delayed peat initiation on emerged landscapes evident since 5 ky cal BP [25] , [26] . Temporal delays in peatland initiation may also be attributed in part to local inundation of the emerging land. The structure of peatland vegetation communities and water table position are tightly coupled, and together control vertical peat growth, C dynamics and the subsequent redistribution of water within the peatland [40] , [42] , [43] . The hydrogeologic setting in the HBL is influenced by regional (for example, 10 2 km 2 ) variability in GIA, and may account for the time lags in peat initiation in our record [25] , [41] . Glaser et al. [25] hypothesize that faster rates of isostatic uplift in downstream reaches compared with corresponding headwaters can reduce slope, impede drainage, re-direct river channels and contribute to anoxic conditions and peatland pattern development in peatlands of the southern HBL [25] , [26] . Our results suggest that similar processes occur across the HBL, whereby the main environmental factor driving the initiation and development of peatlands is the sustained occurrence of waterlogged soils [1] , [25] , [26] . In addition, pond development behind beach ridges during progressive shoreline retreat or winter ice scour in emerging high-energy coastlines, and forest formation on beach ridge before peat initiation, as a consequence of regional isostatic uplift dynamics, are further evidence of the HBL’s dynamic landscape [7] , [9] , [25] , [26] . Thus, the ecological response to hydrogeologic variability can delay paludification of available land and/or terrestrialization of lakes and ponds. Previous global peatland syntheses indicate that the period of most intense northern peatland initiation has been driven by optimal climatic conditions, including high insolation and seasonality, during the early Holocene [15] , [24] , [44] . By contrast, comparisons with available paleoclimate reconstructions reveal an opposite trend in the HBL, such that the most intense period of peatland initiation in the HBL occurred under less favourable conditions. A regional (northern Quebec, Canada) pollen-derived temperature and precipitation reconstruction [29] indicate small climatic anomalies relative to modern climate in the HBL during the Holocene, with the warmest period occurring before land emergence from the Tyrrell Sea. Consequently, all peat initiation and expansion in the HBL progressed under conditions of decreasing summer insolation, increasing winter insolation ( Fig. 2 ), and declining seasonality as inferred from summer–winter insolation differences. In contrast to the warm climate and high summer insolation that supported rapid peat initiation in other northern peatlands during the early Holocene [11] , [15] , maximum rates of peat initiation in the HBL occurred when the climate was coldest and driest ( Fig. 2 ). Although it is possible that peat initiation and expansion may have occurred more rapidly in the HBL under optimal climatic conditions, as it did elsewhere in the early Holocene [15] , the tight coupling between land emergence and peat initiation under cooler/drier mid-Holocene climatic conditions does not appear to have substantively limited the timing or rate of peat initiation. Since 3.5 ky cal BP, peat initiation in the HBL remained relatively low, consistent with declining rates of Neoglacial peat initiation for northern peatlands [15] , [24] . However, declining rates of peat initiation in the HBL occurred under comparatively warmer and wetter conditions relative to the mid-Holocene HBL climate [29] . Examination of North American pollen records of peatland indicators reveals a climatic optimum for peatland extent characterized by a MAT between −2 and 6 °C and mean total annual precipitation (MAP) between 630 and 1,300 mm (ref. 45 ). Further evidence from the West Siberian Lowlands indicates that maximum peatland extent and C pools occur in association with a MAT of 0 °C, which may be a potential climatic optimum for maximizing the difference between net primary production and decomposition [42] , [46] , [47] . Modern climate across most of the HBL falls within these boundary conditions. Thus, in spite of some documented paleoclimatic variability in the HBL [30] , [37] , [48] , peatland development has proceeded within climatic boundary conditions for northern peat initiation and expansion for much of the peat record. Further, on-going rapid land emergence, which results in a lowering of the regional hydraulic gradient, reduced drainage and sustained waterlogged soil conditions, may mask the impact of climatic variation on peatland dynamics in the HBL. Hence, the weaker relationship between climate and peat initiation and expansion in the HBL may be accounted for by a limited ability to consider paleoclimatic variation spatially, and a lack of evidence in support of wide temporal variation in climate at the landscape scale in the HBL. Anticipated high-latitude warming may increase peatland primary productivity and C storage; however, enhanced hydroclimatic variability and intensified land use may augment peatland C decomposition and CO 2 /CH 4 emissions, and result in a positive feedback to climatic warming. Future climate scenarios for the HBL indicate a 2–5 °C temperature increase over the next century, with a concomitant increase in precipitation of 10–15% (ref. 49 ). The implications of these projections may be that warmer, wetter conditions and a longer growing season in the HBL may support continued peatland development and sustained C sequestration via enhanced primary productivity [50] . However, results from a multi-year investigation concerning water balance thresholds in the northern HBL provide confounding evidence, whereby the predicted precipitation increases over the next century in the HBL may not be sufficient to offset the growing season water deficit potential brought about by increasing temperatures and enhanced evaporation [51] . Therefore, disproportionate future temperature increases relative to concomitant precipitation increases may result in reduced peatland C storage capacity in the HBL, with C losses potentially exacerbated by increased fire risk associated with net drier conditions [11] or enhanced anthropogenic activity, such as infrastructure development [52] . Hence, further examination of the spatio-temporal relationship between paleoclimate and C dynamics is warranted, and may reveal a dynamic coupling between the two processes, as it has elsewhere [50] . Based upon new detailed records of peat age and areal C mass, we estimate that the HBL currently stores ~30 Pg C, equivalent to approximately 20% of the North American peatland C pool [41] or approximately 6% of the northern peatland C pool [11] . Although our synthesis includes C data for a range of forested and non-forested bog and fen features, we recognize that the C mass contribution from small bog/fen pools, permafrost features and densely forested peatlands may be under- or over-represented in our C pool estimate, and this requires additional investigation. Although refined estimates of land cover and C mass are needed in the HBL, our evidence provides the most comprehensive synoptic assessment of the modern HBL C pool and demonstrates that the HBL represents a globally significant C sink, underscoring its importance in regional and global C assessments. Still, three decades of peatland CH 4 emission measurements have shown that modern HBL peatlands can be persistent sources of CH 4 to the atmosphere [32] , [33] , [34] , [35] , at a range of spatio-temporal scales. Peatlands release CH 4 to the atmosphere by ebullition, diffusion and plant-mediated transport; however, potential flux estimates are subject to both spatial and temporal uncertainty, due in part to probable nonlinear feedbacks among potential controls over peatland CH 4 flux [13] , [43] . Complex patterns and large ranges (at least 1–50 g CH 4 m −2 y −1 ) in contemporary CH 4 emissions in the HBL have been variously explained by a combination of moderate water table position, gradients in growing seasonal temperatures and heterogeneities in water chemistry and vegetative cover [31] , [32] , [33] , [34] . Consequently, important sources of CH 4 emissions in the HBL have been reported from wet minerotrophic and oligotrophic peatlands, wetlands at the aquatic–terrestrial interface and young coastal fens [31] , [32] , [33] , [53] , [54] . However, recent evidence suggests that CH 4 fluxes from shallow coastal systems may be suppressed by sulfur-rich marine sediments in brackish environments, depending in part upon the vegetation community present [27] , [28] . Thus, the potential for sulfur-mediated CH 4 suppression is recognized here in relation to young or early emerging peatlands. Similarly, landscape-scale assessments using aircraft and surface measurements, together with a chemical transport model, indicate that the inland HBL may release peatland-derived CH 4 at twice the rate of the HBL’s coastal regions [35] , [36] . Accordingly, modern CH 4 emissions from the coastal region of the HBL reportedly range between 5 and 10 g CH 4 m −2 y −1 , whereas the CH 4 emission from the inland peatlands of the HBL range between 15 and 20 g CH 4 m −2 y −1 . Owing to the unique geographic setting of this region in a zone of rapid isostatic uplift and the fact that emerging peatlands pass through a salt marsh or marine-influenced phase, this modern evidence supports our hypothesis that maximum CH 4 flux from HBL peatlands is related to the development of the peat mass rather than simply peat initiation [25] , [37] . Although estimates of CH 4 flux from peatlands to the atmosphere can be highly dynamic, the possible connection between HBL peatland development and potential CH 4 emissions can be evaluated using comparisons between HBL initiation histories and inferred potential CH 4 fluxes ( Fig. 2 ). Peatland development, rather than simply initiation, has been proposed to explain the relationship between CH 4 flux and peat development in the early Holocene [15] , [16] , [24] , [39] . In the HBL, we find that during the most intense period of peat initiation, around 5.5 ky cal BP, the landscape could potentially support CH 4 emissions of 0.7–3.7 Tg CH 4 per year from minerotrophic peatlands and pre-cursor marsh conditions, the occurrence of which is evidenced by reconstruction of past environments following examination of testate amoebae, plant macrofossils and pollen [25] , [26] , [37] , [48] . However, colder, drier conditions during the mid-Holocene together with a possible biogeochemical connection between shallow peat and the underlying marine sediments likely limited the CH 4 flux to the lower end of the range. Temporal lags in peat initiation relative to land availability observed after 5 ky cal BP, coupled with expansion and patterning of peatlands with C-rich pools could further contribute to enhanced peat-derived CH 4 from the HBL to the late Holocene atmosphere, owing to decomposition of both new and old peat [13] , [23] , [55] . Therefore, following several millennia of peatland expansion, a 3-ky cal BP HBL landscape could have potentially contributed 1.2–6.8 Tg CH 4 per year to the late Holocene atmosphere, from the widespread minerotrophic to oligotrophic peatlands [9] , [25] , [32] that were functioning under climatic condition similar to today. Our late Holocene estimates of CH 4 emissions are comparable to those reported using an Earth system modelling approach [2] , [19] , [56] . Using a modelling approach, the HBL was predicted to release ~5 Tg CH 4 per year, which is equivalent to ~10% of the boreal CH 4 emissions [2] , [35] . Further, modelled CH 4 emissions for the broader Hudson Bay region, which includes the HBL as defined here and the adjacent upland region on the Precambrian Shield, suggest a mean snow-free emission of 1.6 Tg CH 4 per year for the period 6 ky cal BP to pre-industrial levels [2] , [19] , [56] . In addition, model evidence used to examine the mid-Holocene decline in CH 4 emissions associated with the 8.2 ky cal BP event, which further confirmed a slight increase in CH 4 emissions from the newly emerging HBL peatlands, at a time when reduced CH 4 emissions from northern peatlands were predicted in response to prevailing cooler/drier climatic conditions [19] . Considered alone, the potential CH 4 fluxes from the HBL are small on a global scale. Although acknowledging the contributions from other biospheric CH 4 sources to late Holocene atmospheric CH 4 dynamics, including tropical wet ecosystems and early anthropogenic activity, our estimates of potential CH 4 flux do convey the role of the HBL in CH 4 accounting. We suggest that a contribution from this large region, together with global peatlands, to atmospheric CH 4 dynamics cannot be ignored. In conclusion, our findings confirm that the most intense period of peat initiation in the HBL occurred during the mid-Holocene, when the climate was colder and received less precipitation than today ( Fig. 2c ) [29] and insolation was decreasing relative to the early Holocene ( Fig. 2a ) [57] . Although climatic conditions in the HBL remained suitable for peat initiation through the mid- to late Holocene, evidence from our study reveals a tight coupling between rapid land emergence from the Tyrrell Sea and peat initiation, as a consequence of GIA. The rate of isostatic uplift varies spatially across the HBL resulting in dynamic hydrogeologic conditions, and suggests that the mid-Holocene delay in peat initiation relative to apparent land emergence may be attributed to localized inundation of the land surface. Based upon new detailed records of peat C density, we estimate that the HBL currently stores ~30 Pg C, which is equivalent to ~20% of the North American [41] or ~6% of the northern C pool [11] . The highest rate of peat initiation in the HBL occurred before the late Holocene rise in atmospheric CH 4 inferred from ice-cores. Using modern regional estimates of snow-free CH 4 flux from the HBL, scaled to a mid- and late Holocene HBL landscape, we further estimate a potential late Holocene CH 4 flux of 1–7 Tg CH 4 per year. This value represents a small but important potential CH 4 emission, when compared with the 21–43 Tg CH 4 per year released by modern northern wetlands [17] . Increased drought frequency and severity are anticipated at many high-latitude peatlands [1] , [24] . However, future climate scenarios predict that the HBL may experience a warmer and wetter climate over the next century [49] , permitting the region to continue to function as a long-term C sink. Nevertheless, disproportionate hydroclimatic change and intensified anthropogenic pressure could decouple the peatland water balance in the HBL, reduce peatland C storage capacity and result in a positive feedback to climatic warming. Improved quantification of modern peatland C stores and regional controls on Holocene peatland C dynamics in the HBL will reduce the uncertainty surrounding the sensitivity of northern peatland C pools under future climate scenarios. Data synthesis and new peat records We compiled 100 records of peat initiation ( Supplementary Table 1 ) from peat profiles located within the physiographic region of the HBL ( Fig. 1 ), spatially defined according to the North American Environmental Atlas [58] . The records were compiled for the purpose of examining the temporal pattern of peatland initiation ( Fig. 2 ) in relation to summer and winter insolation at 60° N (ref. 57 ), variability in ice-core inferred Holocene atmospheric CH 4 (ref. 20 ) and CO 2 (ref. 59 ), post-glacial land emergence [4] , and pollen-reconstructed Holocene temperature and precipitation for the northern Quebec, Canada ecoregion [29] . The northern Quebec ecoregion was selected for the inferred paleoclimate of the HBL because of its proximal location east of Hudson Bay, within a similar bio-climatic setting to the HBL, and having a similar paleoclimatic reconstruction to that produced from a pollen record of a lake core retrieved in the northeastern HBL [30] , [60] . Land emergence, area expansion and the 5.5- and 3-ky shorelines were extracted from the 0.5-ky resolution paleotopography data set [4] , [61] . Peatland area extent and peat thickness were quantified to estimate the potential CH 4 contribution from the HBL to the mid- and late Holocene atmosphere, using previously reported snow-free CH 4 emissions for the HBL [35] . The reported range used here was informed by both static chamber and airborne CH 4 flux measurements. A literature search and a radiocarbon database were used to prepare the synthesis of all available basal dated peat records from the HBL [41] , [62] ( Supplementary Table 1 and original references listed therein), yielding 67 peat records meeting the following three criteria: location (geographic coordinates) within the physiographic region of the HBL; availability of 14 C basal peat ages obtained from the peat–mineral interface; and basal peat material sampled from an ecosystem currently classified as a peatland. To supplement the series of 67 records, field sampling across the Ontario portion of the HBL in 2009–2011 resulted in our contribution of 33 new peat records. Basal dates for the 33 newly sampled peat cores were obtained using accelerator mass spectroscopy 14 C dating of plant remains of known provenance and/or root-free bulk peat ( n <8) at the Keck-CCAMS facility (Irvine, CA, USA), the UGAMS facility (Athens, GA, USA) or Beta Analytic, Inc. (Miami, USA). In the absence of time-weighted peat accumulation rates, paleo-peat thickness was estimated using linear accumulation following peat inception ( n =100); however, we acknowledge that the rate of peat accumulation may vary through time in the HBL. Holocene peat initiation and C dynamics All dates compiled from previous studies, together with the newly dated samples described above, were calibrated using IntCal09 calibration curve [63] in the clam package for R [64] . All calibrated most probable (median) ages are expressed as calendar years before present (1,000 cal y BP=1 ky cal BP), where BP is equal to AD 1950. Although a histogram approach can be problematic when using calibrated radiocarbon dates spanning a probability distribution of >200 years, we selected a bin size equal to the mean 2 σ age uncertainty range of the calibrated radiocarbon dates considered in this study. Each date is represented by a single occurrence in the histogram, and is plotted at the location on the x axis of the median calibrated initiation age [41] . Similar to other studies, we repeated the initiation age binning process using several different numerical approaches and bin sizes (100–500 y) and found that the major trends appeared to be insensitive to the length of time used [21] . Assessment of the lag between peat initiation and land emergence in the HBL was accomplished by spatially relating each peat age in our record with the corresponding time of land emergence. Using the geographic coordinates for each peat record, the corresponding time of land emergence for that location was extracted from the paleotopography data set [4] , [61] . Quantification of the total C pool was based upon bulk density, loss-on-ignition and C content measurements, using standard methods [11] , [65] , on 33 peat cores retrieved during our 2009–2011 field seasons, together with a re-interpretation of seven author-contributed raw data sets from previously published studies [37] , [48] , [52] , [66] , [67] . Direct measurements of C content using homogenized subsamples spanning 4–10 cm of core depth were completed using an ElementarVariomax CN analyzer (Elementar Analysensysteme GmbH, Hanau, Germany). The summed product of incremental bulk density (g cm −3 ) and peat depth (cm) resulted in the areal dry peat mass (g cm −2 ) term. Similar to other studies, areal dry peat mass for the peat profiles examined here was strongly related to basal peat age [68] , [69] . Here, we expressed areal dry peat mass as areal C mass (kg m −2 ), as it was similarly correlated with peat age. Linear regression analysis of C mass and basal peat age revealed a significant relationship (F=41.52; R =0.75, P <0.001, n =36) described by equation (1): Equation (1) was used to estimate areal C mass for the remaining 62 peat cores that lacked reported peat physical properties. The total C pool for the HBL was quantified by multiplying the mean C mass ( n =100) by the total peatland area. C pools for the inland and coastal areas were also calculated separately using mean C masses for these respective regions. The total C pool range was expressed in terms of the 2 σ age uncertainty. Finally, the mean post-initiation C accumulation rate for each sample was calculated by dividing the total peat C pool by the age of the sample and expressed as g C m −2 y −1 . How to cite this article: Packalen, M. S. et al. Carbon storage and potential methane production in the Hudson Bay Lowlands since mid-Holocene peat initiation. Nat. Commun. 5:4078 doi: 10.1038/ncomms5078 (2014).